Membrane curvature sensing by the C-terminal domain of complexin Complexin functions at presynaptic nerve terminals to inhibit spontaneous SNARE-mediated synaptic vesicle (SV) exocytosis, while enhancing stimulated neurotransmitter release. The C-terminal domain (CTD) of complexin is essential for its inhibitory function and has been implicated in localizing complexin to SVs via direct membrane interactions. Here we show that complexin’s CTD is highly sensitive to membrane curvature, which it senses via tandem motifs, a C-terminal motif containing a mix of bulky hydrophobic and positively charged residues, and an adjacent amphipathic region that can bind membranes in either a disordered or a helical conformation. Helix formation requires membrane packing defects found on highly curved membrane surfaces. Mutations that disrupt helix formation without disrupting membrane binding compromise complexin’s inhibitory function in vivo . Thus, this membrane curvature-dependent conformational transition, combined with curvature-sensitive binding by the adjacent C-terminal motif, constitute a novel mechanism for activating complexin’s inhibitory function on the surface of SVs. Complexins are a family of highly conserved cytoplasmic proteins that regulate the synaptic vesicle (SV) fusion machinery and whose expression levels are altered in a variety of neurological and psychiatric disorders [1] , [2] . The precise functions of complexins remain controversial as they are able to both facilitate and inhibit vesicle fusion both in vivo and in vitro . In general, though, it appears that complexin facilitates evoked fusion while inhibiting/clamping spontaneous fusion in worm, fly and mouse neurons; as such, complexin is particularly important for the maintenance of low rates of spontaneous SV exocytosis [2] , [3] , [4] , [5] , [6] , [7] , [8] , [9] , [10] , [11] , [12] , [13] , [14] , [15] , [16] , [17] , [18] . Complexins contain four distinct domains with discrete functions in vesicle fusion: a disordered N-terminal domain that facilitates release [19] , [20] , an inhibitory accessory helix domain [19] , [21] , [22] , [23] , [24] , [25] , [26] , a central helix that binds to the SNARE complex in the groove between synaptobrevin 2 and syntaxin 1 and is essential for all complexin functions [19] , [27] , [28] , [29] , and a disordered C-terminal domain (CTD) that is required for complexin’s inhibition of spontaneous SV exocytosis [3] , [4] , [5] . The complexin CTD was recently shown to bind synthetic phospholipid vesicles, and this complexin–membrane interaction appears necessary for inhibition of spontaneous SV fusion [4] , [30] . Localization of complexin to SVs via CTD–membrane interactions was hypothesized to position complexin to rapidly intercept and clamp assembling SNARE complexes. A conserved amphipathic region of the complexin CTD mediates phospholipid binding for both mammalian and worm complexins, but a novel lipid-binding motif at the very C-terminus of worm complexin was additionally shown to be critical for membrane binding and for complexin’s inhibitory function in C. elegans [4] . Interestingly, a number of complexin isoforms contain a prenylated C-terminal CAAX box motif that mediates membrane binding and that is also essential for the inhibition of spontaneous fusion in some cases [2] , [5] , [6] , [31] , [32] . It remains unclear, however, why complexin might bind to SVs instead of other cellular membranes. What factors draw complexin specifically to SVs? The structure of the protein in the bound state, the energetics of the complexin/membrane interaction and the contributions of lipid composition and topography to binding remain unknown. A distinguishing feature of SVs is their small size and concomitant high surface curvature [33] . Protein motifs such as BAR domains and amphipathic lipid-packing sensor motifs are capable of sensing and/or generating membrane curvature. Surface-associated amphipathic helices (AHs) may sense curvature by responding to the ability of the membrane outer leaflet to accommodate their partial insertion [34] , [35] , [36] , [37] , [38] , [39] , [40] , [41] . Protein sequences containing bulky hydrophobic residues, such as the effector domain of myristoylated alanine-rich C-kinase substrate (MARCKS peptide) also exhibit curvature-dependent membrane interactions [42] . Here we report that the CTD of worm complexin binds to membranes in a curvature-dependent manner. CTD curvature sensing is mediated by two regions, one employing an AH and one employing a MARCKS peptide-like sequence rich in bulky hydrophobic residues. Intriguingly, although the affinity of both motifs for membranes is curvature dependent, the AH motif binds to lower-curvature membranes in a disordered conformation and only adopts a helical structure when bound to ‘accommodating’ membranes such as highly curved vesicles or bilayers with a high degree of acyl chain disorder. Mutations that interfere with helix formation compromise complexin’s function in living worms, indicating that this disorder-to-helix transition is important for proper complexin function on SVs in vivo . The complexin CTD senses membrane curvature Both worm and mammalian complexin interact with synthetic liposomes via a conserved amphipathic motif in the CTD [4] , [30] . Worm complexin was additionally shown to contain a novel lipid binding motif at its very C-terminus that was essential for the complexin–membrane interaction ( Fig. 1a ). Although SV membranes have been proposed as the relevant in vivo binding target, little is known about why complexin might bind SVs selectively. To assess the lipid determinants of membrane binding by worm complexin, we studied its interaction with vesicles of different size and composition using solution state nuclear magnetic resonance (NMR). Proton-nitrogen correlation spectra of wild-type (WT) full-length complexin exhibit intensity decreases (without significant resonance broadening) for a subset of resonances in the presence of liposomes. Residues that are tightly associated with the vesicle exhibit complete signal attenuation in the slowly tumbling bound state, whereas non-interacting residues retain the mobility of the dynamic free state and the consequent high signal intensity. This approach can reliably characterize protein membrane interactions [43] , including those of disordered proteins such as α-synuclein [44] , [45] , [46] , [47] , and yields results that are consistent with more traditional methods such as co-floatation or sedimentation [4] . Thus, equilibrium partitioning of complexin into a lipid-bound state can be probed in a site-specific manner. 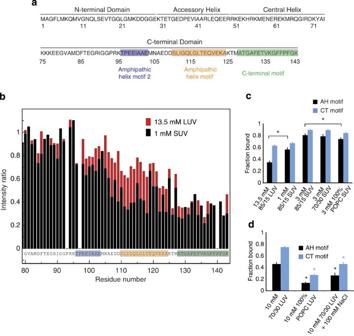Figure 1: Membrane binding by the complexin CTD is curvature dependent. (a) Sequence of worm complexin highlighting three discrete motifs in the CTD: the C-terminal motif (CT motif, green), the amphipathic motif (AH motif, orange) and the second amphipathic motif (AH2, blue). (b) NMR intensity ratios (the ratio of resonance intensity in the presence of vesicles to that in their absence) for 100 μM full-length WT worm complexin in the presence of 13.5 mM LUV lipids (red) and 1 mM SUV lipids (black) in 100 mM NaCl. (c) The average bound fraction of residues in the AH motif (residues 110–124) and CT motif (residues 128–143) of 100 μM full-length WT worm complexin for 85/15 POPC/POPS LUVs compared with SUVs at different concentrations and of different compositions. Black asterisks denote a significant difference (P<0.01,n=15). Differences between LUV and 1 mM SUV for CT motif, between 3 mM 85/15 SUV and 3 mM 70/30 SUV for the AH motif, and between any of the 3 mM SUV CT motif data are not significant (n=15). (d) Bound fraction of the AH and CT motifs of 75 μM full-length WT worm complexin for 70/30 POPC/POPS LUVs in negligible salt compared with LUVs of different compositions and at higher salt concentrations. Black/blue asterisks denote a significant difference (P<0.01) from the 10 mM 70/30 LUV AH (black,n=14) or CT (blue,n=15) motif. Figure 1: Membrane binding by the complexin CTD is curvature dependent. ( a ) Sequence of worm complexin highlighting three discrete motifs in the CTD: the C-terminal motif (CT motif, green), the amphipathic motif (AH motif, orange) and the second amphipathic motif (AH2, blue). ( b ) NMR intensity ratios (the ratio of resonance intensity in the presence of vesicles to that in their absence) for 100 μM full-length WT worm complexin in the presence of 13.5 mM LUV lipids (red) and 1 mM SUV lipids (black) in 100 mM NaCl. ( c ) The average bound fraction of residues in the AH motif (residues 110–124) and CT motif (residues 128–143) of 100 μM full-length WT worm complexin for 85/15 POPC/POPS LUVs compared with SUVs at different concentrations and of different compositions. Black asterisks denote a significant difference ( P <0.01, n =15). Differences between LUV and 1 mM SUV for CT motif, between 3 mM 85/15 SUV and 3 mM 70/30 SUV for the AH motif, and between any of the 3 mM SUV CT motif data are not significant ( n =15). ( d ) Bound fraction of the AH and CT motifs of 75 μM full-length WT worm complexin for 70/30 POPC/POPS LUVs in negligible salt compared with LUVs of different compositions and at higher salt concentrations. Black/blue asterisks denote a significant difference ( P <0.01) from the 10 mM 70/30 LUV AH (black, n =14) or CT (blue, n =15) motif. Full size image Prior work on the interaction of worm complexin with membranes examined binding to large unilamellar vesicles (LUVs) [4] . To examine the role that vesicle size (and thus vesicle curvature) play in complexin liposome binding, we assessed binding to comparably composed (85/15 POPC/POPS) large versus small unilamellar vesicles (SUVs) of ~120 nm and ~30 nm diameter, respectively (as assessed by dynamic light scattering, Supplementary Fig. 1A ). The complexin CTD binds to both LUVs and SUVs in a dose-dependent manner ( Fig. 1b and Supplementary Fig. 1B ). With LUVs, the C-terminal ~15 residues (128–143) bind most strongly, with segments at increasing distance from the C-terminus displaying diminishing interactions. Upon addition of SUVs, however, uniform binding of a larger C-terminal stretch of ~35 residues is observed, with strong signal attenuation extending all the way to residue 110 in the N-terminal direction, unlike with LUVs. Significant albeit weaker binding is additionally observed for residues 95–109. For 85/15 POPC/POPS vesicles in 100 mM NaCl, more than a tenfold higher concentration of LUVs is required to achieve binding comparable to that observed with SUVs for the C-terminal residues ( Fig. 1b,c ). Thus, complexin clearly shows a higher affinity for the more highly curved SUVs. Importantly, we observe similar CTD membrane binding and curvature sensitivity for mouse complexin ( Supplementary Fig. 2 ), and membrane binding by the mouse complexin CTD was also recently shown to be critical for its inhibitory function [9] . These data demonstrate that complexin’s CTD binds more readily to more highly curved membrane surfaces. SVs, at approximately 30–40 nm diameter, present a much more highly curved membrane surface than the plasma membrane and are comparable in size to the SUVs used here [33] . As such, membrane curvature may play a key role in selective localization of complexin to SVs. To explore the role of electrostatic versus hydrophobic interactions in complexin binding to vesicles of different sizes, we generated both negatively charged POPC/POPS and neutral POPC-only vesicles. For LUVs, elimination of negative vesicle charge substantially diminished binding throughout the C-terminus ( Fig. 1d and Supplementary Fig. 1C ); this implies that electrostatics play an important role in binding to these less highly curved vesicles. Likewise, the presence of 100 mM NaCl impairs binding to LUVs compared with binding in the absence of salt ( Fig. 1d ). Surprisingly, binding to SUVs was nearly unaffected by vesicle charge and was comparable for both neutral POPC-only and negatively charged POPC/POPS membranes with either 15 or 30% POPS ( Fig. 1c and Supplementary Fig. 1C ). These results suggest that electrostatics play a less significant role in CTD binding to SUVs, compared with LUVs. Accordingly, the interaction of the CTD with highly curved vesicle membranes is likely dominated by hydrophobic interactions between membrane-inserted apolar residues and lipid acyl chains. The CTD binds highly curved membranes via distinct motifs Prior analyses of complexin CTD sequences identified a potential AH sequence spanning residues approximately 116–133. Experimentally, a corresponding but slightly shifted amphipathic region comprised of residues 110–124 (AH motif) was observed to bind LUVs weakly, whereas a novel C-terminal lipid-binding motif (CT motif) spanning the very C-terminal ~15 residues (128–143) binds LUVs tightly [4] . To explore the importance of these motifs for binding to highly curved membranes, we analysed binding curves from SUV-into-protein NMR titrations ( Supplementary Fig. 3 and Supplementary Table 1 ). The two motifs exhibit different binding properties, with an apparent SUV lipid affinity of 7 μM for the CT motif and 19 μM for the AH motif. We further characterized SUV binding by two mutants that target the CT and AH motifs and were previously demonstrated to perturb LUV binding and to eliminate complexin’s inhibitory function in vivo [4] . Deletion of the C-terminal 12 residues (Δ12 mutant) abolished binding of complexin to SUVs ( Fig. 2 and Supplementary Fig. 1D ) indicating that the CT motif is essential for binding highly curved membranes. Upon replacement of hydrophobic AH motif residues L117 and V121 with glutamate (LV/EE mutant), SUV binding of the AH motif is disrupted but binding of the CT motif is unperturbed ( Fig. 2 and Supplementary Fig. 1D ). Thus, the CT motif binds membranes independently of the AH motif and the two motifs are distinct. Interestingly, in the LV/EE mutant, AH motif residues C-terminal to the V121E mutation retain a significant degree of membrane binding ( Supplementary Fig. 1D ), indicating that binding of the AH motif is not cooperative across the entire motif. 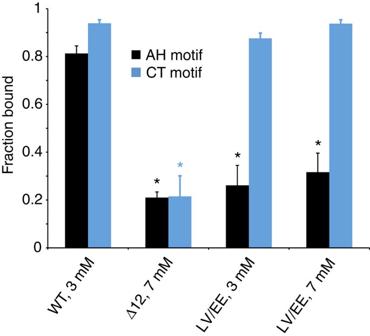Figure 2: Deletion of the CT motif or mutation of the AH motif impairs membrane binding. Bound fractions of the AH and CT motifs for WT, Δ12 and LV/EE complexin. Binding of both motifs is eliminated for the Δ12 mutant, but only binding of the AH motif is eliminated for the LV/EE mutant. Proteins used at a concentration of 100 μM. Black/blue asterisks denote a significant difference (P<0.01) from the WT AH (black,n=15,11,11,11) or CT (blue,n=15,3,15,15) motif. Figure 2: Deletion of the CT motif or mutation of the AH motif impairs membrane binding. Bound fractions of the AH and CT motifs for WT, Δ12 and LV/EE complexin. Binding of both motifs is eliminated for the Δ12 mutant, but only binding of the AH motif is eliminated for the LV/EE mutant. Proteins used at a concentration of 100 μM. Black/blue asterisks denote a significant difference ( P <0.01) from the WT AH (black, n =15,11,11,11) or CT (blue, n =15,3,15,15) motif. Full size image A detailed analysis of the structural propensities of the CTD of worm complexin based on NMR chemical shifts, relaxation rates and nuclear Overhauser effects (NOEs; Supplementary Note and Supplementary Fig. 4 ) reveals that AH motif exhibits a slight, but detectable, preference for helical structure even in the absence of membranes, whereas the CT motif does not exhibit any secondary structure preferences, further demonstrating that these motifs possess distinct and independent structural properties. Interestingly, a region of the CTD N-terminal to the AH motif (residues 96–104), which we term the AH2 motif, exhibits a strong signature for helical structure ( Supplementary Fig. 4 ). The AH motif binds SUVs but not LUVs in a helix conformation Although the AH motif was identified based on its potential for forming AH structure and displays weak helical character in lipid-free complexin ( Supplementary Note and Supplementary Fig. 4 ), it remains unclear whether this region folds into a helix upon membrane binding. To address this, we turned to circular dichroism (CD) spectroscopy to examine secondary structure changes upon membrane binding. The CD spectrum of free complexin contains minima at ~204 and ~222 nm, consistent with a mix of helical and random coil structure ( Fig. 3a ). Addition of SUVs led to a dose-dependent increase in negative ellipticity at 222 nm ( Fig. 3a,b ), indicating that SUV-binding induces helical structure. Comparable spectral changes were observed upon addition of SUVs to a truncated complexin fragment consisting of only the CTD (residues 91–143), demonstrating that the helical structure occurs within the CTD ( Fig. 3c ). Unexpectedly, addition of LUVs to complexin (either full-length or the truncated CTD construct) under conditions where NMR shows that both the CT and AH motifs are bound did not alter the CD spectra ( Fig. 3a,c ), indicating that the CTD binds to less highly curved vesicles in a conformation devoid of secondary structure. 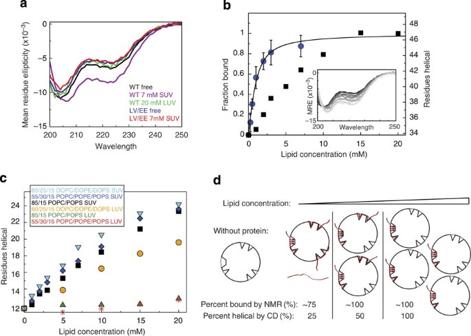Figure 3: Helix formation by the amphipathic helical (AH) motif requires membrane defects. (a) CD spectra of 100 μM WT and LV/EE full-length complexin in the absence/presence of SUVs and LUVs. Increased helicity is observed only for the WT protein with SUVs. (b) Comparison of membrane binding, as observed by NMR (circles), with helix formation, as observed by the CD signal at 222 nm (squares), at increasing SUV concentrations with 100 μM full-length WT complexin. [θ]222was used to estimate the number of helical residues. Individual spectra shown in the inset (0–20 mM lipid from black to light grey). (c) Helix formation by the isolated complexin CTD (residues 91–143) plotted as the number of helical residues estimated using [θ]222, (see Methods) at increasing concentrations of: 85/15 POPC/POPS LUVs (green triangles), 85/15 POPC/POPS SUVs (black squares), 60/25/15 DOPC/DOPE/DOPS LUVs (orange circles), 60/25/15 DOPC/DOPE/DOPS SUVs (cyan triangles), 55/30/15 POPC/POPE/POPS LUVs (red stars) and 55/30/15 POPC/POPE/POPS SUVs (blue diamonds). Helix formation occurs only for SUVs or for LUVs containing dioleoyl lipids. (d) Schematic model for saturable helix formation by the AH motif upon addition of SUVs. SUVs are depicted with multiple small defects capable of binding disordered protein regions and a single larger defect capable of binding an AH. Note that defects likely form dynamically41, and should not be considered as stable features. As noted in the text, it appears that highly curved vesicles can form/accommodate a limited number of defects extensive enough to accommodate helix formation by the AH motif. At the lowest depicted SUV concentration, most of the protein (two out of four depicted molecules) is bound to the smaller defects in a disordered conformation and only a small amount (one out of four molecules) can bind in a helical conformation, whereas the remainder (one out of four molecules) remains unbound. At double the SUV concentration, all of the protein can bind, but only half (two of four depicted molecules) can bind in a helical conformation, whereas the other half can only bind in a disordered conformation. Doubling the SUV concentration again allows all of the protein molecules to bind in a helical conformation. Figure 3: Helix formation by the amphipathic helical (AH) motif requires membrane defects. ( a ) CD spectra of 100 μM WT and LV/EE full-length complexin in the absence/presence of SUVs and LUVs. Increased helicity is observed only for the WT protein with SUVs. ( b ) Comparison of membrane binding, as observed by NMR (circles), with helix formation, as observed by the CD signal at 222 nm (squares), at increasing SUV concentrations with 100 μM full-length WT complexin. [θ] 222 was used to estimate the number of helical residues. Individual spectra shown in the inset (0–20 mM lipid from black to light grey). ( c ) Helix formation by the isolated complexin CTD (residues 91–143) plotted as the number of helical residues estimated using [θ] 222 , (see Methods) at increasing concentrations of: 85/15 POPC/POPS LUVs (green triangles), 85/15 POPC/POPS SUVs (black squares), 60/25/15 DOPC/DOPE/DOPS LUVs (orange circles), 60/25/15 DOPC/DOPE/DOPS SUVs (cyan triangles), 55/30/15 POPC/POPE/POPS LUVs (red stars) and 55/30/15 POPC/POPE/POPS SUVs (blue diamonds). Helix formation occurs only for SUVs or for LUVs containing dioleoyl lipids. ( d ) Schematic model for saturable helix formation by the AH motif upon addition of SUVs. SUVs are depicted with multiple small defects capable of binding disordered protein regions and a single larger defect capable of binding an AH. Note that defects likely form dynamically [41] , and should not be considered as stable features. As noted in the text, it appears that highly curved vesicles can form/accommodate a limited number of defects extensive enough to accommodate helix formation by the AH motif. At the lowest depicted SUV concentration, most of the protein (two out of four depicted molecules) is bound to the smaller defects in a disordered conformation and only a small amount (one out of four molecules) can bind in a helical conformation, whereas the remainder (one out of four molecules) remains unbound. At double the SUV concentration, all of the protein can bind, but only half (two of four depicted molecules) can bind in a helical conformation, whereas the other half can only bind in a disordered conformation. Doubling the SUV concentration again allows all of the protein molecules to bind in a helical conformation. Full size image The CD spectrum of the LV/EE complexin mutant showed no change upon addition of SUV concentrations that elicited a large increase in helicity for the WT protein ( Fig. 3a ). Given the location of the LV/EE mutation within the AH motif, this observation indicates that the helical structure induced in WT complexin upon binding to SUVs results from folding of the AH motif. Supporting this assertion, the increased CD signal at 222 nm upon SUV binding corresponds to approximately 13 residues forming helical structure ( Fig. 3b,c ), in reasonable agreement with the length of the AH motif (15 residues). Helix formation requires saturable SUV-binding sites To investigate the basis for helix formation by the AH motif, we compared the accrual of helical structure (monitored by CD) with membrane binding (monitored by NMR) at increasing SUV lipid concentration ( Fig. 3b ). The data reveal that binding of the AH motif is complete at lipid concentrations where helix formation is far from complete. Thus, the AH motif can exist in an unstructured SUV-bound conformation, which converts to the helical state only upon addition of more SUVs. The most parsimonious explanation for this observation is that SUVs have a limited capacity for binding the AH motif in a helical conformation, compared with binding in unstructured conformations. AHs are known to require significant accommodation, often described in terms of sites of exposure of the hydrophobic membrane interior (so called packing defects), by the membrane bilayer upon binding [34] , [35] , [36] , [38] , [39] , [41] . SUVs may be able to accommodate or dynamically form a limited number of sites/packing defects extensive enough to bind the AH motif in a helical conformation. The formation of less extensive SUV sites/defects that can bind the AH motif in an unstructured form may be less restricted. Thus, adding more SUVs increases the number of helix-binding sites and enables more of the protein to convert from the bound, but unstructured, conformation (reported on by NMR) to the bound helical conformation (reported on by CD). This interpretation, illustrated schematically in Fig. 3d , would also account for the non-hyperbolic shape of the CD-binding curve ( Fig. 3b ). Increased LUV acyl chain disorder enables helix formation If packing defects of a particular extent or type are required to bind the AH motif in a helical conformation, we reasoned that making LUVs more accommodating to helix insertion by altering their lipid composition could allow some degree of helix formation by the AH motif. Indeed, LUVs formed using dioleoyl instead of palmitoyl-oleoyl acyl chains (composition 60/25/15 DOPC/DOPE/DOPS), expected to facilitate membrane insertion at the acyl chain level because of increased acyl chain disorder [48] , resulted in the accrual of substantial helical structure in the CTD with increasing LUV lipid concentration ( Fig. 3c ). In contrast, replacement of 30% of the POPC by the smaller-headgroup ‘conical’ phospholipid POPE, expected to create space and facilitate membrane insertion at the headgroup level [48] did not result in any helix formation upon CTD binding to LUVs ( Fig. 3c ). Thus, it appears that helix formation by the AH motif requires insertion into and perturbation of the acyl chain region of the bilayer, and that highly curved membranes such as SUVs are able to accommodate such insertion at a limited number of sites/packing defects per vesicle, whereas LUVs with a physiological membrane composition do not readily accommodate such insertion. SV-like composition does not alter helix formation SV membranes contain a very high proportion of unsaturated acyl chains [33] , but binding to SUVs composed of dioleoyl lipids (60/25/15 DOPC/DOPE/DOPS) did not result in further increase in helix formation in the complexin CTD over that observed with palmitoyl-oleoyl lipids ( Fig. 3c and Supplementary Fig. 5 ). SVs also contain a substantial amount of cholesterol, which can alter membrane properties, but binding to SUVs composed of dioleoyl lipids plus 40% cholesterol (36/15/9/40 DOPC/DOPE/DOPS/cholesterol) did not alter helix formation in complexin’s CTD ( Supplementary Fig. 5 ). Thus, helix formation by the AH motif persists upon binding to SUVs that more faithfully approximate the composition of SVs. Helix formation is necessary for inhibitory function in vivo To explore whether helix formation by the AH motif, rather than membrane binding alone, is important for complexin function, we sought mutations that preserve binding but interfere with helix formation by the AH motif. We identified two mutants, K123P and Q114P/E119P, that show unperturbed SUV binding of the AH motif by NMR ( Fig. 4a ), but exhibited marked decreases in SUV-induced helicity by CD ( Fig. 4b ). Both of these mutations compromise complexin’s inhibitory function in worms ( Fig. 4c ; previously shown for K123P) [4] , and the rank order of the effect on function in vivo ( Fig. 4d ) is the same as that on helicity in vitro ( Fig. 4b ). These results imply that helix formation specifically, rather than just membrane binding, by the AH motif is important for complexin’s inhibitory function. 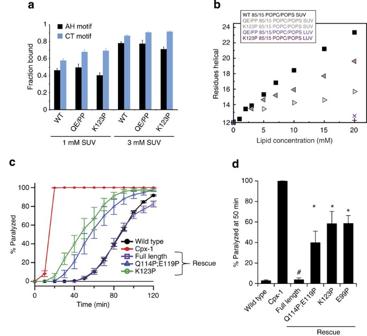Figure 4: Helicity in the AH and AH2 motifs is important for complexin’s inhibitory function. (a) The bound fraction of residues, as determined by NMR, in the AH motif (residues 110–124) and CT motif (residues 128–143) for WT, Q114P/E119P and K123P truncated complexin (CTD construct, residues 91–143) in the presence of 1 and 3 mM 85/15 POPC/POPS SUVs. Differences between any of the 1 mM SUV or 3 mM SUV AH data are not significant (n=14–16). (b) Helix formation, plotted as the number of helical residues estimated using [θ]222(see Methods) for WT, Q114P/E119P and K123P truncated complexin (CTD construct, residues 91–143) in increasing concentrations of 85/15 POPC/POPS SUVs or LUVs: WT with SUVs (black squares), Q114P/E119P with SUVs (beige left triangles), K123P with SUVs (grey right triangles), Q114P/E119P with LUVs (purple X) and K123P with LUVs (maroon plus) (c) Paralysis time course on 1 mM aldicarb for WT (black),cpx-1mutant (red), full-length CPX-GFP rescue (purple), K123P CPX-GFP rescue (green) and Q114P/E119P CPX-GFP rescue (blue) animals. (d) Percentage of animals paralysed on 1 mM aldicarb after 50 min for WT,cpx-1mutant and transgenic animals expressing complexin variants as indicated. Aldicarb data for K123P were reported previously4. *A significant difference (P<0.01) from both WT andcpx-1and#no significant difference from WT (n=163(wt),35(cpx1),16(fl),11(QE/PP),21(K123P),10(E99P). Figure 4: Helicity in the AH and AH2 motifs is important for complexin’s inhibitory function. ( a ) The bound fraction of residues, as determined by NMR, in the AH motif (residues 110–124) and CT motif (residues 128–143) for WT, Q114P/E119P and K123P truncated complexin (CTD construct, residues 91–143) in the presence of 1 and 3 mM 85/15 POPC/POPS SUVs. Differences between any of the 1 mM SUV or 3 mM SUV AH data are not significant ( n =14–16). ( b ) Helix formation, plotted as the number of helical residues estimated using [θ] 222 (see Methods) for WT, Q114P/E119P and K123P truncated complexin (CTD construct, residues 91–143) in increasing concentrations of 85/15 POPC/POPS SUVs or LUVs: WT with SUVs (black squares), Q114P/E119P with SUVs (beige left triangles), K123P with SUVs (grey right triangles), Q114P/E119P with LUVs (purple X) and K123P with LUVs (maroon plus) ( c ) Paralysis time course on 1 mM aldicarb for WT (black), cpx-1 mutant (red), full-length CPX-GFP rescue (purple), K123P CPX-GFP rescue (green) and Q114P/E119P CPX-GFP rescue (blue) animals. ( d ) Percentage of animals paralysed on 1 mM aldicarb after 50 min for WT, cpx-1 mutant and transgenic animals expressing complexin variants as indicated. Aldicarb data for K123P were reported previously [4] . *A significant difference ( P <0.01) from both WT and cpx-1 and # no significant difference from WT ( n =163(wt),35(cpx1),16(fl),11(QE/PP),21(K123P),10(E99P). Full size image The mechanisms by which helix formation by the AH motif mediate complexin function are presently unclear. We noted that the AH2 motif, located N-terminal to the AH motif in the worm complexin CTD ( Fig. 1a and Supplementary Fig. 4B ), exhibits a significant degree of membrane binding to SUVs but not LUVs ( Supplementary Fig. 1B ), which is eliminated by the LV/EE mutation ( Supplementary Fig. 1D ), suggesting that it depends on helix formation by the AH motif. Thus, helix formation by the AH motif may mediate functionally relevant changes in other complexin regions, such as the AH2 motif. To directly test the functional importance of the AH2 motif, we designed a mutation to interrupt its helical character by introducing a proline at position 99. Intriguingly, this mutation significantly compromises complexin’s inhibitory function ( Fig. 4d ). We have demonstrated that the complexin CTD binds preferentially to highly curved membranes and senses membrane curvature via tandem lipid binding motifs: a C-terminal motif (residues 128–143) and an upstream amphipathic motif (residues 110–124; Fig. 1 ), providing a potential mechanism for selective binding to SVs versus the plasma membrane or other less highly curved cellular membranes. The binding of each of the CT and AH motif exhibits curvature sensitivity, and a simplistic analysis of their NMR-derived binding curves suggests that binding by each requires accommodation by the membrane and that an increase in binding sites/packing defects as a function of increasing curvature is primarily responsible for their curvature sensitivity ( Supplementary Note , Supplementary Fig. 3 and Supplementary Table 1 ). Both the CT and the AH motif bind initially via conformations that are devoid of secondary structure, as monitored by CD, but the AH motif folds into a helical structure when bound to membranes that are highly curved (that is, SUVs) or rich in unsaturated acyl chains. A growing number of membrane surface-associated proteins have been identified as sensors and/or modulators of membrane curvature, but the mechanistic basis for curvature sensing remains an active area of research. Some proteins employ shape complementarity to recognize curved membrane. Examples include BAR domains, which form a crescent-shaped surface that recognizes (and may also impose) a specific degree of membrane curvature [35] , [40] , [49] . Other mechanisms rely on membrane properties that result from curvature, rather than on the explicit geometrical curvature of the membrane. A common example involves the insertion of AHs (noting that insertion here does not mean transmembrane insertion). It is generally agreed that such insertion requires lateral displacement of both lipid headgroups and acyl chains in the outer leaflet of the membrane to sterically accommodate burial of the apolar face of the helix in the interior of the membrane [35] , [36] , [37] , [38] , [39] , [41] . Positive curvature is thought to strain the ability of the outer leaflet to maintain optimal headgroup and acyl chain packing and thereby facilitate the accommodation of AH insertion at resulting packing defects. The most critical mediator of membrane binding by complexin is the CT motif, as its deletion completely abrogates membrane binding ( Fig. 2 ), and also completely eliminates complexin’s inhibitory function in living worms [4] . Unlike the AH motif, the CT motif does not form secondary structure in the bound state for any condition examined here. Nevertheless, binding of the CT motif is clearly and strongly dependent on membrane curvature ( Fig. 1 , Supplementary Fig. 3A and Supplementary Table 1 ), with an order of magnitude increase in apparent affinity for SUVs versus LUVs. The 16-residue CT motif contains four phenyalanine residues, which are known to contribute to the binding of other peptide sequences to membranes by inserting into the hydrophobic membrane interior. The best characterized example of this is the MARCKS peptide, which contains 5 phenylalanines in a span of 25 residues that contribute significantly to the energetics of MARCKS membrane binding [50] , [51] , [52] , [53] , [54] . Furthermore, like the CT motif of complexin, MARCKS has recently been shown to bind selectively to highly curved membranes in an unstructured conformation in a manner that critically depends on its phenylalanines [42] . Thus, in a manner analogous to that discussed above for AHs, the insertion of bulky phenylalanine residues into membranes also appears to require some degree of accommodation, or packing defect, which is facilitated by positive membrane curvature. This effect is the likely origin of curvature sensing by the CT motif of complexin. Notably, the CT motif also contains two positively charged lysines, which might be expected to confer affinity for negatively charged membranes, but this is a much lower positive charge density when compared with the 12 lysines and 1 arginine in MARCKS. Accordingly, binding of the CT motif to SUVs is dominated by the hydrophobic effect (sequestration of phenylalanine side chains in membrane interior; Fig. 1c ). The AH motif of complexin binds to membranes more weakly than the CT motif. In the absence of the CT motif, no significant AH motif binding is observed under our conditions in vitro , but when anchored near the membrane by the adjacent CT motif, the AH motif clearly associates with the membrane surface ( Figs 1 and 2 ). Like the CT motif, the AH motif binds to LUVs in an unstructured conformation ( Fig. 3 ). Because the AH motif contains no phenylalanines, it is likely that the partitioning of other hydrophobic side chains within the motif into the hydrophobic membrane region mediates membrane association. This is supported by the observation that eliminating two hydrophobic side chains via the LV/EE mutation greatly reduces LUV [4] and SUV ( Fig. 2 ) binding by the AH motif. As for the CT motif, such binding is inherently curvature dependent because membrane insertion requires accommodation by packing defects, which is facilitated by positive curvature. In the presence of SUVs, the AH motif binds initially in a disordered conformation but undergoes a saturable conformational transition to a helical conformation ( Fig. 3 ). This conformation is likely favoured both by the amphipathic nature of the motif as well as by its weak preference for helical conformations even in the absence of membranes ( Supplementary Fig. 4 and Supplementary Note ). Although helix formation can also occur upon replacement of saturated lipid acyl chains with unsaturated acyl chains in LUVs, such lipids are rare in vivo , and it is thus likely that the AH motif only samples helical conformations when the protein is bound to very highly curved membranes such as SVs. Thus, helix formation by the AH motif adds a second layer of curvature sensitivity, which appears to operate like a binary switch rather than via the rheostat-like tuning of binding affinity exhibited by more typical curvature-sensing AHs. The two-step binding behaviour we observe for the AH motif has been predicted by computational simulations of the binding and folding of endophilin’s H0 AH to membranes of different curvature [41] . H0 was observed to fold into a helix upon binding to membranes of high curvature, but unstructured bound states were also observed in the simulations. Binding to planar membranes occurred only via unstructured conformations. This behaviour may be common for the binding of AHs to membrane surfaces, but the bound-yet-disordered conformation is not typically observed, probably because it converts rapidly to the helical conformation if possible or dissociates rapidly if not. Indeed, for H0, the bound state is always observed experimentally to be helical [38] , [55] , and experimental observations of bound but disordered states have never been reported. It is also interesting to compare the behaviour of the AH motif with the curvature-sensitive AH formed by the SV-binding protein α-synuclein. Despite a paucity of bulky apolar residues, hydrophobicity plays a significant role in synuclein membrane binding, and accordingly synuclein also binds preferentially to sites of membrane packing defects [34] , [56] , [57] . Unlike the AH motif, however, the binding of synuclein to negatively charged SUVs features a strong electrostatic contribution from a plethora of positively charged residues [47] , [58] , [59] , [60] . This enables synuclein to bind to negatively charged membranes even in the absence of packing defects. Indeed, synuclein binds to lower curvature vesicles, albeit with a lower affinity [47] , [58] , [59] , [61] , and it is possible that synuclein may interact with the plasma membrane directly [62] . Despite a significant electrostatic contribution to its membrane affinity, no observations of bound but disordered states of synuclein have been reported. In the case of complexin, it appears that the membrane-bound CT motif keeps the AH motif near the membrane surface, effectively increasing its local concentration and generating a detectable population of the bound-yet-disordered state when conversion to the helical state is not possible. Thus, our observations of the AH motif uniquely recapitulate the simulated binding process, lending support to both the simulation and our results. Sequence analysis indicates that the AH motif in worm complexin is likely conserved across species and mediates membrane binding in mammalian complexins as well [4] , [30] . The predicted AH motif of mammalian complexin-1 was previously shown to bind to membranes [30] , and we have shown here that it binds preferentially to highly curved membranes. Thus, it appears likely that the presence and behaviour of the AH motif is general to all complexins. In contrast, the CT motif region of complexin is more divergent. Many complexins (for example, squid, leech and variants of fly and mammalian complexins) contain a C-terminal CAAX box, and farnesylation of this CAAX box motif likely mediates membrane association for these variants [5] , [6] . Like mammalian complexin-1 and -2, worm complexin does not feature a CAAX box and instead binds to membranes at its C-terminus via the CT motif [4] . Our data for mouse complexin-1 ( Supplementary Fig. 2 ) demonstrate membrane binding by its C-terminal residues as well. Thus, membrane binding at the C-terminus of complexin, mediated either by prenylation or by motifs such as the worm complexin CT motif, appears to be a highly conserved feature of the protein. We have shown here that membrane binding by the worm complexin CT motif is highly sensitive to membrane curvature and have shown that this holds for mammalian complexin-1 as well, suggesting that curvature sensing is conserved for CT motifs of non-CAAX box complexins. Because lipid-modified proteins have been shown to sense membrane curvature in a packing defect-dependent manner [39] , it is possible that C-terminally farnesylated complexins also prefer highly curved membranes and localize to SVs. Notably, mammalian complexin-3 and -4 were shown to localize strongly and specifically to presynaptic terminals, which contain highly curved SVs, and not to bouton-free axonal regions, which are bounded by the relatively flat plasma membrane [63] . Furthermore, fly complexin also localizes to presynaptic terminals when expressed in mouse neurons [5] and the Drosophila complexin CAAX box was shown to be necessary for inhibition of spontaneous exocytosis at the fly neuromuscular junction [5] , [6] , consistent with our own work showing that binding of worm complexin to SVs is essential for the inhibition of spontaneous exocytosis [4] . Clearly, further studies are needed to compare the membrane-binding behaviours of CAAX box containing and CAAX box-free complexins, but the data available suggest that binding to highly curved vesicles could well be a conserved feature of both. We recently demonstrated that localization of worm complexin to SVs via its CTD was necessary for the inhibition of spontaneous exocytosis [4] . Here we have shown that the CTD, in addition to mediating complexin’s membrane binding, confers curvature sensitivity to this binding. Although a growing number of protein motifs are capable of sensing membrane curvature, complexin is apparently unique in that it contains tandem lipid-binding motifs with distinct binding and sensing properties. The CT motif discriminates between different membrane curvatures through enhanced affinity for more highly curved membranes. This undoubtedly increases the population of synaptic-vesicle bound complexin, but cannot prevent some population of complexin bound to other membranes. Indeed, depending on the relative surface area of SV membranes versus other membranes, a considerable population of complexin could bind to the plasma membrane or other cellular membranes. In contrast to the CT motif, the AH motif binds to membranes with a relatively weak affinity, and is unable to localize complexin to membranes in the absence of the CT motif. Although binding of the AH motif also exhibits some degree of curvature sensitivity, the more dramatic response of the AH motif to highly curved membranes is its conversion from an unstructured conformation to a helical structure. This conversion is strongly dependent on membrane curvature, and indeed only occurs for very highly curved membranes such as SV-sized liposomes. A fourfold increase in vesicle diameter completely abrogates this structural transition ( Fig. 3 ). Thus, the helical conformation of the AH motif is unlikely to be found on any cellular membranes other than SVs or comparably curved membrane structures. As localization of complexin to SVs is required for its inhibitory function, and the CT and AH motif act in concert to generate a SV-specific state of complexin, it is reasonable to posit that this state is functional with respect to inhibition of SNARE-mediated vesicle fusion. At present, it is not clear why a helical conformation of the AH motif would confer function. One possibility is that helix formation increases the residence time of complexin on membranes, and this increases the efficiency with which complexin can intercept and clamp zippering SNARE complexes. A second possibility is that helix formation by the AH motif is important for facilitating functional protein–protein interactions, either directly or via structural orchestration of other complexin regions such as the upstream AH2 motif. Notably, a complexin region upstream of the mouse AH motif has been proposed to form functional interactions with synaptotagmin [64] , the critical SV-localized calcium sensor for SNARE-mediated synaptic transmission. Thus, complexin interactions either with synaptotagmin or other SV proteins (including possibly complexin itself) could depend on helix formation by the AH motif, which in turn occurs only when complexin is bound to SVs. Localization of complexin to SVs is critical for its inhibitory function [4] . We have now shown that the membrane-binding CTD of complexin exhibits a marked preference for highly curved membrane surfaces that is mediated by a pair of tandem membrane-binding motifs. A C-terminal motif confers increased affinity for highly curved membranes, likely by inserting phenylalanyine side chains into the membrane interior; this requires accommodating sites/packing defects in the membrane that are formed more easily and in greater numbers for positively curved membranes. An upstream amphipathic motif binds to membranes initially in an unbound conformation, likely through similar insertion of hydrophobic side chains. This motif can undergo a transition into a helical structure only when bound to very highly curved membranes that favour AH insertion, presumably at larger accommodation sites/packing defects. We hypothesize that although the C-terminal motif favours binding of complexin to SVs versus other cellular membranes, the formation of a helical conformation by the amphipathic motif serves as a gating mechanism for activating complexin’s inhibitory function only when the protein is bound to the surface of SVs ( Fig. 5 ). This represents a unique and novel mechanism of curvature sensing and SV localization. 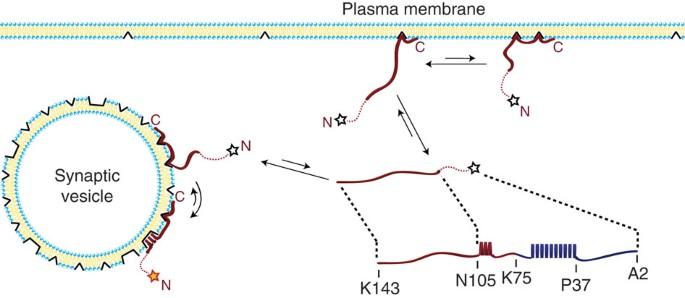Figure 5: The CT and AH motif combine to localize and gate complexin function on SVs. The CT motif, spanning residues 128–143 binds membranes in an unstructured conformation through insertion of hydrophobic phenylalanine residues at small packing defects. An increased density of such packing defects on highly curved membranes confers an increased affinity for highly curved SVs. The AH motif, spanning residues 110–124, also binds membranes in an initially unstructured conformation through insertion of hydrophobic side chains. In the presence of larger packing defects, found only on highly curved membranes, the AH motif can convert into a helical structure. The inhibitory function of complexin is only activated (red/orange star) upon helix formation by the AH motif. When the AH motif is unstructured, complexin’s inhibitory function is inactivated (empty stars). Complexin thus employs rheostat-like binding by the CT motif to preferentially localize the protein to SVs combined with a binary switch-like helical folding transition of the AH motif to gate its inhibitory function only at the SV surface. Figure 5: The CT and AH motif combine to localize and gate complexin function on SVs. The CT motif, spanning residues 128–143 binds membranes in an unstructured conformation through insertion of hydrophobic phenylalanine residues at small packing defects. An increased density of such packing defects on highly curved membranes confers an increased affinity for highly curved SVs. The AH motif, spanning residues 110–124, also binds membranes in an initially unstructured conformation through insertion of hydrophobic side chains. In the presence of larger packing defects, found only on highly curved membranes, the AH motif can convert into a helical structure. The inhibitory function of complexin is only activated (red/orange star) upon helix formation by the AH motif. When the AH motif is unstructured, complexin’s inhibitory function is inactivated (empty stars). Complexin thus employs rheostat-like binding by the CT motif to preferentially localize the protein to SVs combined with a binary switch-like helical folding transition of the AH motif to gate its inhibitory function only at the SV surface. Full size image Protein purification Worm complexin WT, complexin CTD fragment (residues 91–143) and mouse complexin-1 were cloned into the pET SUMO vector with no additional sequence tags. The L117E/V121E (LV/EE), K123P and Q114P/E119P (QE/PP) mutants were generated via site-directed mutagenesis of the WT construct. The Δ12 mutant was generated by inserting a stop codon at position 132. The full-length WT protein was used in all experiments except where explicitly noted. Proteins were expressed in bacterial cultures and purified as previously described [4] . Briefly, BL21(DE3) Escherichia coli cells were transformed with the relevant plasmid and grown in Luria-Bertani media to an optical density of ~0.6. To produce unlabelled protein, cells were induced with isopropyl-β- D -thiogalactoside (IPTG) and grown for 3–4 h before collection. To produce 15 N and 15 N 13 C isotopically labelled protein, cells were pelleted, washed and transferred to minimal media containing 15 N-labelled ammonium chloride or both 15 N-labelled ammonium chloride and 13 C-labelled glucose before induction with IPTG for 3–4 h. All worm complexins lacked the N-terminal methionine, whereas mouse complexin-1 contained all residues. Cells were lysed by sonication on ice, supernatants were clarified by centrifugation at 40,000 r.p.m. for 45 min, and SUMO-tagged fusion protein was purified from supernatants on a Ni-NTA column and dialyzed into 20 mM Tris pH 8, 150 mM NaCl, 1 mM dithiothreitol. The His 6 -SUMO affinity tag was cleaved by SUMO protease and purified complexin was isolated through a second run over a Ni-NTA column. Protein was dialysed into distilled water, frozen and lyophilized. Similar NMR heteronuclear single quantum coherence (HSQC) spectra and comparable lipid-binding behaviour were observed for lyophilized protein versus protein directly dialysed into buffer. To prepare deuterated protein for the transferred NOE experiments, cells were grown directly in minimal media made in D 2 O and containing 15 N ammonium chloride to an optical density of 0.6 and induced with IPTG for 3–4 h. For NMR, lyophilized protein was dissolved in 60 mM phosphate (or 50 mM PIPES) pH 6.1, 2 mM dithiothreitol, 0.5 mM EDTA, with 100 mM NaCl except where explicitly noted. For CD, lyophilized protein was dissolved in 20 mM phosphate pH 6.1, 100 mM NaCl, 0.5 mM EDTA. Protein concentration was estimated by absorbance at 280 nm using an extinction coefficient of 1,490 M −1 cm −1 , or for quantitative binding curves, by comparing Coomassie-stained gel band intensities for complexin dilutions with a set of BSA standards. Liposome preparation Lipids were obtained from Avanti Polar Lipids and stored at −20 °C. Lipids were mixed and dried under N 2 gas and residual solvent was removed under vacuum for 1 h. After resuspension in buffer, LUVs were prepared by ten cycles of freezing in liquid nitrogen and thawing in warm water followed by repetitive extrusion through 400 nm and then 100 nm pore-size polycarbonate films (21 times each) using a 1-ml Avanti Mini-Extruder from Avanti Polar Lipids [4] . For SUVs, lipids were mixed and dried as above, resuspended, subjected to bath sonication for 3 × 5 min and further clarified by centrifugation at 60,000 r.p.m. for 2 h. Vesicle size and purity were verified by dynamic light scattering for both SUV and LUV preparations on multiple occasions. Vesicles were stored at 4 °C and used within 1 week. Lipid concentration was estimated based on the amounts of starting lipid, but for quantitative binding curves, lipid concentration was determined using a phosphate quantification assay. Briefly, lipid samples (or sodium phosphate standards) were treated with perchloric acid and heated to 150° for 1 h. After addition of ammonium molybdate and ascorbic acid, samples were heated for 10 min at 100°. Absorbance at 797 nm was measured, and lipid concentrations were obtained through comparison to phosphate standards. NMR spectroscopy Mouse complexin-1 resonance assignments were transferred directly from Fig. 2 in Pabst et al . [28] Worm complexin assignments were transferred from previously published assignments of His-tagged complexin [4] and confirmed/corrected using additional heteronuclear triple resonance three-dimensional spectra (HNCACB, and HNCACO/HNCO) obtained for untagged WT and LV/EE worm complexin on a Bruker AVANCE 800 MHz spectrometer equipped with a cryoprobe (New York Structural Biology Center). Complete assignments were obtained for backbone carbonyl carbons, backbone amide groups, and α- and β-carbons, excepting the two N-terminal residues and a poorly resolved stretch from residues 46 to 63. For the K123P and QP/EE mutants, assignments could be reliably transferred for all resonances save those in the AH motif region, which shifted too much to transfer residue-specific assignments. However, the intensity ratio analysis of the AH motif as a whole could still be carried out for these mutants using the average intensity for the shifted, unassigned resonances. Proton-nitrogen heteronuclear correlation spectra (HSQC spectra) used for intensity ratio analysis were obtained on either a Varian Unity Inova 600 MHz spectrometer equipped with a cryoprobe or on a Bruker AVANCE 500 MHz spectrometer equipped with a room temperature probe. Typical spectral widths and number of complex data points in each dimension were 20 p.p.m./1,024 points for 1H, 23.5 p.p.m./80–256 points for 15 N dimension, 15 p.p.m./80 points for CO and 75 p.p.m./150 points for Cα/β. Data were referenced indirectly to 4,4-dimethyl-4-silapentane-1-sulfonic acid (DSS) and ammonia based on the position of the water resonance [65] . Random coil values obtained from linear hexapeptides in 1 M urea at pH 5.0 and 25 °C (ref. 66 ) were used to calculate Cα-Cβ secondary shifts. Free state and SUV-bound R2 relaxation experiments were performed on a Bruker AVANCE 800 MHz spectrometer equipped with a cryoprobe (New York Structural Biology Center) using a Car-Purcel-Meiboom-Gill (CPMG) pulse sequence with 900 μs between Pi pulses and relaxation delays of 16.96, 33.92, 50.88, 67.84, 84.8, 101.76, 135.68, 169.6, 203.52, 237.44, 271.36, 305.28 and 339.2 ms. Additional free state and SUV- or LUV-bound R2 relaxation experiments were performed on a Varian Unity Inova 600 MHz spectrometer equipped with a cryoprobe using a CPMG pulse sequence with 625 μs between pi pulses and relaxation delays of 10, 30, 50, 70, 90, 130, 170 and 210 ms. SUV- and LUV-bound HSQC-NOE SpectroscopY-Transverse Relaxation Optimized SpectroscopY (HSQC-NOESY-TROSY) experiments were performed using 15N-labelled, deuterated protein on a Bruker AVANCE 900 MHz spectrometer equipped with a cryoprobe (New York Structural Biology Center), whereas equivalent spectra for free protein were obtained on a Bruker AVANCE 800 MHz spectrometer equipped with a cryoprobe (New York Structural Biology Center). Free state spectral widths were 23 p.p.m. in both indirect dimensions and 12 p.p.m. in the direct dimension. Complex data points of 50, 50 and 1,024 were collected for the two indirect and the direct dimensions, respectively. For LUV- and SUV-bound spectra, spectral widths were 22 p.p.m. in both indirect dimensions and 12 p.p.m. in the direct dimension. With LUVs, 48 complex data points were collected in both indirect dimensions, whereas 1,024 complex data points were collected in the direct dimension; for SUVs, 48 and 40 complex data points were collected in each indirect dimension, with 1,024 points collected for the direct dimension. CD spectroscopy Far-ultraviolet CD spectroscopy experiments were performed on an AVIV Biomedical Model 410 CD Spectrometer. CD spectra were obtained from 200 to 250 nm at 25 °C with a wavelength step of 1 nm, an averaging time of 1.7 s, and with three or four averaged scans per sample. A cell path length of 0.02 cm was used, with protein concentrations typically at 75 or 100 μM. Data for the full-length protein were converted to mean residue molar ellipticity and the helicity was estimated using [θ] 222 (ref. 67 ). For the isolated CTD construct, which lacks Tyr and Trp residues, reliable protein concentrations could not be obtained and the CD data were instead normalized so that the estimated helical content in the absence of liposomes matched that predicted for this region based on the NMR data ( Supplementary Note ). Lipid binding data analysis HSQC spectra were acquired with and without liposomes and intensity ratios were calculated on a per-residue basis as cross-peak intensity in the presence of liposomes divided by the free state cross-peak intensity. Intensity ratios directly reflect the fractional population of the unbound state for each residue. The fraction bound of the CT and AH motifs was obtained by averaging the intensity ratio for all residues within each motif, respectively, and subtracting this value from 1. Binding curves were obtained by repeating this analysis at different lipid concentrations. Protein stock concentration was estimated using Coomassie-stained SDS gels by comparison of gel bands with BSA standards. Final protein concentrations are indicated in figure legends and typically ranged from 30 to 100 μM. Lipid concentration was estimated using the phosphate assay described above. Curves were fit using the nonlinear curve-fitting module in XMgrace following the treatment of Pfefferkorn and Lee [68] . Specifically, curves were fit to the equation: where K a app , the apparent association constant, and B max , the maximum binding sites per lipid molecule, are the fit parameters. P t is the total protein concentration and L is the total lipid concentration. The number of lipids per binding site can be calculated as the inverse of B max . Strains Animals were maintained at 20 °C on agar nematode growth media seeded with OP50 bacteria as previously described [69] . Robust synaptic expression of all constructs was verified by measuring synaptic fluorescence as previously described [4] (not shown). Strains in this study include: N2 Bristol and cpx-1(ok1552) . Transgenic strains: JSD291: tauls90;cpx-1 [P snb-1 ::CPX-GFP] Extrachromosomal arrays: JSD216: tauEx55;cpx-1 [Psnb-1::CPX(K123P)-GFP] JSD0739: tauEx259;cpx-1 [Psnb-1::CPX(Q114P;E119P)-GFP] JSD675: tauEx221;cpx-1 [P snb-1 ::CPX(E99P)-GFP] Aldicarb sensitivity assays To measure aldicarb sensitivity, 20–25 young adult animals were placed on agar plates containing 1 mM aldicarb and scored for paralysis at 10 min intervals for 2 h (Chem Services). Each assay contained ten plates of 20–25 animals for each genotype tested. The experimenter was blind to the genotypes. Each genotype was tested at least ten times and paralysis curves were generated by averaging paralysis time courses for each plate [70] . Statistical analysis Student’s t -test was used to compute significance for pairwise comparisons and the Tukey–Kramer method for multiple comparisons. Significance was defined by the criterion P <0.01. Error bars represent ±s.e.m. How to cite this article: Snead, D. et al . Membrane curvature sensing by the C-terminal domain of complexin. Nat. Commun. 5:4955 doi: 10.1038/ncomms5955 (2014).